A carbon nanotube wall membrane for water treatment Various forms of carbon nanotubes have been utilized in water treatment applications. The unique characteristics of carbon nanotubes, however, have not been fully exploited for such applications. Here we exploit the characteristics and corresponding attributes of carbon nanotubes to develop a millimetre-thick ultrafiltration membrane that can provide a water permeability that approaches 30,000 l m −2 h −1 bar −1 , compared with the best water permeability of 2,400 l m −2 h −1 bar −1 reported for carbon nanotube membranes. The developed membrane consists only of vertically aligned carbon nanotube walls that provide 6-nm-wide inner pores and 7-nm-wide outer pores that form between the walls of the carbon nanotubes when the carbon nanotube forest is densified. The experimental results reveal that the permeance increases as the pore size decreases. The carbon nanotube walls of the membrane are observed to impede bacterial adhesion and resist biofilm formation. Carbon nanotubes (CNTs) were recently formed into a nanoporous membrane structure [1] , and molecular transport through the tubes was observed. This vertically aligned CNT membrane with opened CNT tips, known as an open-ended CNT membrane, has since been used in water treatment applications [2] , [3] . At approximately the same time, another type of CNT membrane was introduced [4] , in which the interstices between nanotubes in a vertical array of CNTs were utilized as membrane pores; this membrane is known as an outer-wall CNT membrane [5] , [6] . Fluid flow in CNTs has attracted considerable interest because of the frictionless or near frictionless flow [3] , [7] , [8] , [9] , [10] in CNTs. However, the water permeance through CNT membranes [1] , [2] , [3] was initially not considerably different from that attainable using a commercial polysulfone (PSf) ultrafiltration (UF) membrane [11] , which is approximately several hundred litres per square metre per hour (LMH bar −1 ). Only recently has a water permeability of 2,400 LMH bar −1 been achieved [11] . This permeability is not considerably greater than the permeability that can be attained using non-CNT membranes. However, the observed flow rate in a CNT membrane is several orders of magnitude greater than that predicted by the conventional fluid flow theory [10] . This fact suggests that the permeance through a CNT membrane should and could be substantially enhanced compared with the values reported to date. Vertically grown CNT forests [12] have typically been used as outer-wall CNT membranes. Although water treatment is the primary interest here, the outer-wall membrane is a vertically aligned mesoporous structure. This type of mesoporous structure has received considerable attention because of its strong potential in the fields of catalysis, optics, biosensors and biomolecule separation [13] , [14] . Therefore, the ability to manipulate the structural characteristics of CNT membranes, such as their pore dimensions, pore density and tortuosity, is desirable for various applications. One efficient approach for manipulating such structural characteristics is through densification of the vertically grown CNT forest. Two relatively simple densification methods have been developed: capillary densification [15] and mechanical densification [16] . The capillary densification method is not suitable for this purpose because CNTs collapse and form bundles on densification [15] and cannot be manipulated. By contrast, the mechanical densification method, which involves compressing the CNT forest in the direction perpendicular to the CNT walls, can be used to vary the pore size, for instance, between 7 and 38 nm. In this work, we demonstrate that the water permeability of a CNT membrane can approach 30,000 LMH bar −1 when the CNTs in the membrane are fully utilized in the form of a CNT wall membrane that is well defined and when they are tailored for rapid transport. We first consider the outer-wall membrane, which is then transformed into a CNT wall membrane. Densified CNT array and outer-wall CNT membrane A vertically grown CNT forest and densified CNTs that can be used as outer-wall membranes are shown in Fig. 1a,b , respectively. The vertical CNTs were super-grown using water-assisted chemical vapour deposition (CVD), which extends the lifetime of the catalyst through the use of a moderate oxidant and yields high-density and high-aspect-ratio CNTs (length/CNT inner diameter) [12] . The CNT forest shown in Fig. 1a is 1.3 mm high and vertically aligned on a silicon substrate ( Supplementary Fig. 1a ). A ‘skin layer’ covering the surface, which can block the fluid flow, is not observed in the image of the top surface of the CNT forest ( Supplementary Fig. 1b and 2 ). The average inner diameter and wall number of the CNTs, as statistically measured from high-resolution tunnelling electron microscopy (HR-TEM) images, were 4.8nm and 2.7, respectively, and they were generally Gaussian-distributed ( Supplementary Fig. 3 ), with an aspect ratio of 2.7 × 10 5 (length (1.3 mm)/inner diameter (4.8 × 10 −6 mm)). As shown in the HR-TEM images ( Supplementary Fig. 4a,b ), the vertical CNTs have a bamboo-free structure without the inner wall crossing the inner space of the CNTs; in addition, no catalyst nanoparticles block the inner space [17] . The as-grown vertical CNTs are, on average, approximately several tens of nanometres apart from one another, and thus, the interstices created by the vertical CNTs can be utilized as membrane pores, that is, as an outer-wall CNT membrane. 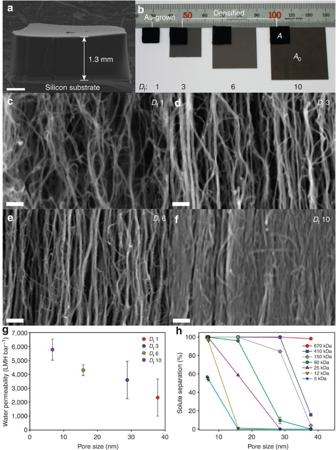Figure 1: Densified CNT array and performance of the outer-wall membrane. (a) SEM image of super-grown CNT forest (scale bar, 500 μm). (b) Optical photographs of densified CNT forests that were used as the outer-wall CNT membranes. TheDfis the ratio of the CNT area before densification to that after densification. The area (A) is 1 cm2for all cases, whereas the area occupied by as-grown CNTs (A0) varies depending on theDfvalue. In the case of aDfof 10, 10 cm2of as-grown CNTs were densified into 1 cm2of compressed CNTs. (c–f) Cross-sectional SEM images (× 300,000 magnification, scale bar, 100 nm) of densified CNTs. GreaterDfvalues indicated that the CNTs were more closely packed and more straightened. The figures present the fracture plane images of the CNT array. (g) Water permeability, as affected by theDffor the outer-wall CNT membrane. Data are shown as the mean±s.d.,n=3 independent outer-wall membranes tested for the permeability measurement. (h) Rate of rejection by the densified outer-wall CNT membranes obtained with seven types of dextran (5–670 kDa). Dextran solutions with a concentration of 100 mg l−1were filtered by the densified outer-wall CNT membrane under a pressure of 1 bar at 20 °C. Figure 1: Densified CNT array and performance of the outer-wall membrane. ( a ) SEM image of super-grown CNT forest (scale bar, 500 μm). ( b ) Optical photographs of densified CNT forests that were used as the outer-wall CNT membranes. The D f is the ratio of the CNT area before densification to that after densification. The area ( A ) is 1 cm 2 for all cases, whereas the area occupied by as-grown CNTs ( A 0 ) varies depending on the D f value. In the case of a D f of 10, 10 cm 2 of as-grown CNTs were densified into 1 cm 2 of compressed CNTs. ( c – f ) Cross-sectional SEM images (× 300,000 magnification, scale bar, 100 nm) of densified CNTs. Greater D f values indicated that the CNTs were more closely packed and more straightened. The figures present the fracture plane images of the CNT array. ( g ) Water permeability, as affected by the D f for the outer-wall CNT membrane. Data are shown as the mean±s.d., n =3 independent outer-wall membranes tested for the permeability measurement. ( h ) Rate of rejection by the densified outer-wall CNT membranes obtained with seven types of dextran (5–670 kDa). Dextran solutions with a concentration of 100 mg l −1 were filtered by the densified outer-wall CNT membrane under a pressure of 1 bar at 20 °C. Full size image The characteristics of the pore structure of the outer-wall CNT membrane, such as its pore dimensions, pore density and pore tortuosity, can be altered and manipulated using the mechanical densification method to obtain better membrane performance or to render the membrane more suitable for use in various applications [16] ( Supplementary Fig. 5 ). Figure 1b presents optical images of densified CNT arrays (outer-wall CNT membranes) that were obtained by compressing the CNTs (grey area in the figure) to a lateral area of 1 cm 2 (black rectangular area in the figure). For convenience, we define the densification factor, D f , as the ratio of the area occupied by CNTs before compression or as-grown CNTs ( A 0 ) to that occupied by compressed CNTs after densification ( A ); thus, a D f ( A 0 / A) value of 10 corresponds to a tenfold densification of the as-grown CNTs. Three densified outer-wall CNT membranes with D f values of 3, 6 and 10 ( Fig. 1b) and one as-grown outer-wall CNT membrane ( D f of 1) were used in the experiments. The cross-sectional scanning electron microscopy (SEM) images presented in Fig. 1c–f show that larger densification factors result in greater densities of the CNTs. The size of the interstitial space between neighbouring CNTs, which is the average pore size in the outer-wall CNT membrane, was measured using the pore-flow solute transport model with dextran [18] , [19] , [20] (see Methods for details). The characteristics of the outer-wall CNT membrane are summarized in Table 1 . The results in this table indicate that the pore size can be controlled from several tens of nanometres, which corresponds to the membrane with a D f of 1, to 6.7 nm, which corresponds to the membrane with a D f of 10. Furthermore, the results in Table 1 also indicate that the pore density can be increased by an order of magnitude—from 8.14 × 10 10 cm −2 ( D f of 1) to 83.3 × 10 10 cm −2 ( D f of 10) as a result of the mechanical densification. Another characteristic of interest for membranes is the tortuosity of the pores, which was statistically measured from high-magnification SEM images. The tortuosity (Γ) was calculated from L e / L , where L is the straight CNT length and L e is the curved CNT length. The results in Table 1 clearly indicate that the tortuosity approaches unity as the densification factor increases, which, in turn, indicates that the CNTs or the pores in the outer-wall membrane can be straightened by the densification. Table 1 Characteristics of the CNT membranes. Full size table These results demonstrate that mechanical densification is a simple yet effective approach for manipulating and altering the membrane characteristics to obtain the desired membrane performance. The process for fabricating the outer-wall CNT membrane is illustrated in Supplementary Fig. 6 . The outer-wall membrane has an area of 1 cm 2 and a thickness of 1.3 mm. Water permeability is well known to decrease as the pore size of the membrane is decreased to remove finer impurities. However, the outer-wall CNT membrane does not follow this well-known behaviour, as revealed by the water permeability plotted in Fig. 1g , which was determined using a dead-end membrane filtration system ( Supplementary Fig. 7 ). This figure clearly shows that the water permeability for the outer-wall CNT membrane increases with decreasing pore size or increasing densification of the CNT array; the water permeability increases from an average of 2,300±1,330 LMH bar −1 for a D f of 1 (as-grown) to an average of 5,800±760 LMH bar −1 for a D f of 10, which is a greater than twofold increase in the permeability as a result of the densification. As shown in Table 1 , the pore size of the membrane decreases with increasing densification, decreasing from 37.8 nm for a D f of 1–6.7 nm for a D f of 10. Taken together, these experimental results clearly reveal the unique feature of the outer-wall membrane, where a smaller membrane pore size leads to greater water permeability, as shown in Fig. 1g . To determine the reason for the enhanced water permeability, we independently obtained the pore area ( Supplementary Note 1 ) and calculated the flow velocity of water from experimentally obtained hourly volumes of purified water. As shown in Table 1 , the flow velocity increased with increasing densification, which is the reason for the increase in water permeability. It is well known that hydrophobic CNT walls lead to a frictionless flow and thus a high flow velocity because of the weak interfacial force between water molecules and atomically smooth, hydrophobic CNT walls [1] , [3] , [10] . Molecular ordering occurring inside of the tube has also been proposed as an explanation of the high flow velocity [21] , [22] , [23] . As the densification increases, more CNT wall surface becomes available for water flow, thereby resulting in a greater velocity. For the unique features of the outer-wall CNT membrane to be valuable, the ability of the membrane to reject finer impurities should still be retained as the pore size is decreased for higher water permeability. To demonstrate the particle rejection behaviour of the outer-wall membranes, experiments were conducted using dextran solutions (100 mg l −1 ) of seven types of dextrans (5, 12, 25, 80, 150, 410 and 670 kDa) under 1 bar of pressure at 20 °C. The rejection rate ( R ) was determined according to the equation ( C f −C p )/ C f × 100, where C f and C p are the feed concentration and the permeate concentration, respectively. Figure 1h presents the rejection rates for the various types of dextran solutions that were achieved by the outer-wall CNT membranes densified to various levels of D f from 1 to 10. This figure clearly indicates that a more densified membrane or a membrane with a smaller pore size removes finer particles. This result experimentally demonstrates that, in this densified outer-wall CNT membrane system, higher water permeability is achieved with a smaller pore size while retaining the ability to remove finer impurities. In this regard, the outer-wall CNT membranes with D f values of 3, 6 and 10 all demonstrated 100% rejection of 670 kDa dextran, indicating that no micron-scale cracks were present in the membranes. The particle rejection ability of the outer-wall membranes with a D f of 10 is comparable to that of a commercial UF membrane ( Supplementary Table 1 ). Some aspects of this CNT membrane could be optimized to obtain better membrane performance. First, the CNT walls can be cleaned to obtain higher water permeability. Many amorphous carbons and defects are known to be present on the outer walls of CVD-grown CNTs [24] . The Raman spectrum of the as-grown CNTs shown in Supplementary Fig. 8 indicates that the peak intensity ratio of the G-band to the D-band ( I G / I D ) is relatively low at 0.93, indicating a high density of amorphous carbon and defects on the outer wall. These amorphous carbons and defects can retard the flow, particularly in the case of highly densified CNTs because of a reduction in available area of smooth CNT surface that enhances the velocity. Thus, removing the amorphous carbon is desirable to increase the velocity. For this purpose, a thermal treatment could be used, particularly given that, in an oxygen atmosphere, the oxidation temperature of amorphous carbon is lower than that of sp 2 -bonded carbon [25] , [26] . To establish a systematic approach to remove the carbon, thermogravimetric analyses were performed, as shown in Supplementary Fig. 9 . This figure shows that the weight loss was only 5% at temperatures up to 600 °C; however, after this temperature was exceeded, a precipitous loss occurred, reaching almost 100% loss at 720 °C. To arrive at an optimal heating schedule, the heating time and the final temperature were varied. The corresponding CNT purity determined from the Raman peak intensity ratio ( I G / I D ) is shown in Supplementary Fig. 8 (ref. 27 ). As shown, heating to 500 °C at a rate of 5 °C min −1 (100 min) yielded the highest intensity ratio; this heat treatment was therefore used to remove amorphous carbon in ambient air. The water permeability through the outer-wall CNT membrane with a D f of 10 before and after the thermal purification of CNTs is shown in Fig. 2 , along with the water permeabilities reported in the literature for other CNT membranes [1] , [2] , [3] , [5] . The water permeability of the outer-wall membrane is observed to have more than double as a result of the heat treatment due to the corresponding increase in the water flow velocity ( Table 1 ). A control experiment was conducted to determine whether rendering the CNT surface hydrophilic reduces the permeability. For this purpose, a pyrenebutyric acid treatment was performed to make the surface hydrophilic [28] . With this treatment, the permeability for the thermally purified outer-wall membrane ( D f of 10) decreased to 5,378 from 13,200 LMH bar −1 . This reduction in permeability can be attributed to the hydrophilicity of the CNT walls, which leads to an enhanced interaction between water molecules and the walls. 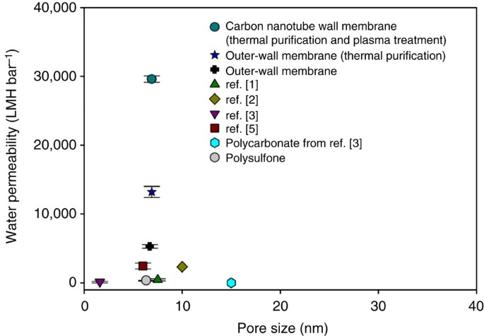Figure 2: Water permeabilities. Water permeabilities obtained in this work and those reported by other researchers in the literature based on CNT membranes. Polycarbonate and polysulfone membranes (UE4040, Woongjin Chem Co.) are commercial membranes. The data obtained in this work are shown as the mean±s.d. forn=3 independent membranes tested for the permeability measurement. Figure 2: Water permeabilities. Water permeabilities obtained in this work and those reported by other researchers in the literature based on CNT membranes. Polycarbonate and polysulfone membranes (UE4040, Woongjin Chem Co.) are commercial membranes. The data obtained in this work are shown as the mean±s.d. for n =3 independent membranes tested for the permeability measurement. Full size image CNT core membrane Another aspect of the CNT membrane that could be exploited to improve membrane performance is the effect of the entrance resistance of the CNT on the water permeability. The authors of an earlier study based on molecular dynamics simulations [22] , [29] reported that a high external pressure (>120 bar at CNT entry, >1,000 bar at CNT exit) is required for water molecules to pass through the inner pores of pristine CNTs with a hydrophobic surface. These theoretical studies suggest that a hydrophilic surface modification should decrease the resistance at the entrance and exit of the pores of hydrophobic CNT membranes. For this purpose, an oxygen plasma treatment in the form of oxygen reactive-ion etching (RIE) was performed on the surface of the outer-wall CNT membrane. Oxygen RIE was chosen to open the CNT fullerene caps to make the inner pores of the CNTs available for water passage during the process of making the entrances and exits of the pores hydrophilic [30] . The formation of hydrophilic functional groups was confirmed using the X-ray photoelectron spectroscopy (XPS), as shown in Supplementary Fig. 10 . We employed micro-Raman spectroscopy to determine whether the RIE also renders the entire membrane surface hydrophilic. The graph for the CNT wall section shows that the I G / I D ratio for the wall section did not change after the treatment ( Supplementary Fig. 11a ). The ratio for the CNT end-cap section, however, decreased from 0.926 to 0.841 ( Supplementary Fig. 11b ). This decrease occurs as a consequence of the introduction of some defects or oxygen-containing functional groups on the CNT end during removal of the cap ( Supplementary Fig. 10b ). The dual effects resulting from the oxygen RIE, that is, opening of sealed CNT tubes and making the entrances hydrophilic, led to a significant increase in the water permeability, as shown in Fig. 2 ; the water permeability increased more than twofold compared with that obtained after thermal treatment. This attained water permeability of the CNT wall membrane, which is close to 30,000 LMH bar −1 , is more than an order of magnitude greater than the highest water permeability reported for CNT membranes ( ∼ 2,400 LMH bar −1 ) [11] . To separate the effect of CNT cap opening from that of rendering the entrances hydrophilic, separate experiments were performed with open-ended CNT membranes; in these experiments, the CNT caps were removed by microtoming (denoted as ‘mechanical’ in Table 1 ). The pores of the open-ended membrane formed by microtoming were observed using HR-TEM ( Supplementary Fig. 12 ). The increase in water permeability because of the oxygen plasma treatment for the same mechanically prepared CNT membranes (second and third rows from the bottom in the table) amounts to 67%, which indicates that rendering the entrances and exits hydrophilic leads to an increase of 67% for the CNT membrane. Given that the permeability increased by a factor of 2.2 as a consequence of the oxygen RIE, the increase in the permeability in multiples that can be attributed to the opening of capped CNT tubes is 1.9. The permeance of the open-ended membrane prepared by O 2 plasma is 1,900 LMH bar −1 (first entry from the bottom in Table 1 ) and that of the open-ended membrane fabricated by microtoming is 2,000 LMH bar −1 (the second entry). From these experimental results, we determined the fraction of open-ended CNTs for the plasma-treated membrane by dividing 1,900 by 2,000, which yields 95% for the fraction of the CNT tips opened by oxygen plasma relative to the microtomed open-ended CNT tips. The assumption here is that all CNT ends were opened by microtoming (the process for fabricating the open-ended CNT membrane by microtoming and that by oxygen RIE are illustrated in Supplementary Figs 13 and 14 , respectively). On the basis of the permeabilities presented in the third entry from the bottom and in the first entry from the top in the table, the multiple is 1.5 ((2,300+0.95 × 1,200)/2,300), which is in good agreement with the independent value of 1.9. The CNT wall membrane exhibits performance similar to that of the outer-wall membrane ( D f of 10 and thermally purified D f of 10) in terms of the ability to reject particles ( Supplementary Table 1 ), despite the significant increase in water permeability. The slip lengths affected by densification and by the thermal and plasma treatments are presented in Supplementary Fig. 15 ( Supplementary Note 1 ). Biofouling characteristics CNT membranes are known to exhibit antibiofouling capability because of their ability to inactivate bacteria. However, in the case of CNT membranes, the effects of biofouling on bacterial adhesion are unknown. To investigate the biofouling behaviour of the outer-wall CNT membrane, bacterial adhesion tests were conducted for 72 h. Pseudomonas aeruginosa PA01 was selected in this study because this species is commonly found in wastewater and is primarily responsible for membrane biofouling [31] , [32] , [33] . Two independent aspects of biofouling are of interest: bacterial adhesion and biofilm formation. To investigate bacterial adhesion, confocal laser scanning microscopy (CLSM) images were examined and compared for various cases, as shown in Fig. 3a,d,g for the outer-wall CNT membrane ( D f of 10), CNT wall membrane and commercial PSf UF membrane, respectively. In these CLSM images, green colour indicates live cells and red colour represents dead cells. After 24 h of testing, fewer cells were observed to have adhered on both CNT membranes compared with the number adhered to the commercial PSf UF membrane, which indicates that the CNT membrane has an antiadhesion property. Interestingly, very few dead cells were observed on the CNT membrane surface. This result demonstrates that the CNT membrane impedes bacterial adhesion, presumably because of its rough surface at the nanoscale. This result reveals another aspect of antibiofouling behaviour that has not previously been observed. The ability of the CNT membrane to impede bacterial adhesion is in contrast to the previously reported antimicrobial properties of CNTs that are ascribed to the sharp edges of CNTs causing physical damage to cell membranes, eventually leading to the inactivation of bacteria [34] , [35] , [36] . 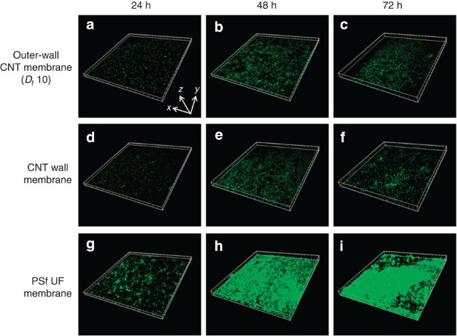Figure 3: Biofouling characteristics of CNT membranes. CLSM images as a function of time: (xaxis: 512 μm,yaxis: 512 μm,zaxis: (a,d,g) 12–14 μm after 24 h, (b,e,h) 20–26 μm after 48 h and (c,f,i) 23–32 μm after 72 h. In the images, live bacteria cells are green and dead cells are red. Figure 3: Biofouling characteristics of CNT membranes. CLSM images as a function of time: ( x axis: 512 μm, y axis: 512 μm, z axis: ( a , d , g ) 12–14 μm after 24 h, ( b , e , h ) 20–26 μm after 48 h and ( c , f , i ) 23–32 μm after 72 h. In the images, live bacteria cells are green and dead cells are red. Full size image The behaviour of P. aeruginosa PA01 biofilm formation that follows the cell adhesion was examined on the basis of the CLSM images obtained after testing for 48 and 72 h; these images are shown in Fig. 3b,e,h and Fig. 3c,f,i , respectively. A clear distinction is observed between biofilm formation on CNT membranes and that on the commercial PSf UF membrane. As evident in Fig. 3i , abundant bacteria adhered on the PSf UF membrane, resulting in the formation of a well-mature biofilm. By contrast, biofilm formation is observed to have progressed considerably less on the outer-wall CNT membranes ( Fig. 3c ) and the CNT wall membrane ( Fig. 3f ). In fact, the concentration of P. aeruginosa PA01 on the CNT membranes after 72 h ( Fig. 3c,f ) appears to be similar to that after 48 h ( Fig. 3b,e ). The better resistance to biofilm formation exhibited by the CNT membranes is a distinct advantage. The densified outer-wall CNT membrane is unique in that a decrease in the pore size of the membrane results in an increase in the water permeability. Another unique feature of the densified outer-wall CNT membrane is that the pore diameter can be readily varied in the range between 7 and 38 nm through simple mechanical compression. This feature would be attractive when the membrane is used as a flexible, vertically aligned mesoporous material for potential applications in catalysis, sorption, gas sensing, optics, photovoltaics and macromolecule separation, including protein separation. The CNT wall membrane that can be obtained by thermal and oxygen-plasma treatments of the densified outer-wall membrane represents a new class of membrane. It can deliver a water purification capacity that exceeds that of any CNT membrane by more than an order of magnitude, reaching a level of 30,000 LMH at 1 bar, which is almost two orders of magnitude greater than that attainable using traditional polymer membranes. The antibiofouling capability of the CNT wall membrane is considerably enhanced by its ability to impede bacterial adhesion, in addition to its capability to resist biofilm formation. CNT synthesis and characterization Vertically aligned CNTs were synthesized using water-assisted CVD in a horizontal quartz tube furnace with an inner diameter of 4 inches. Layers of 1-nm-thick Fe and 20-nm-thick Al were deposited on a silicon (Si) substrate using an e-beam evaporator and sputter. The substrate area (A 0 ) for the open-ended CNT membrane and those for D f values of 1, 3, 6 and 10 were 0.5 × 0.5, 1 × 1, 1.8 × 1.8, 2.5 × 2.5 and 3.2 × 3.2 cm 2 , respectively. The CNTs were grown in a quartz tube at 810 °C (using a ramp rate of 810 °C min −1 ) for 16 min with C 2 H 2 (210 s.c.c.m.) as the carbon source, Ar (480 s.c.c.m.) as the carrier gas and H 2 O vapour (generated by bubbling Ar at 222 s.c.c.m. through water at 60 °C) as a growth enhancer. All gases were simultaneously introduced into the tube at the beginning of the growth process. The CNTs that were separated from the substrate were weighed using a Sartorius BT 224S balance. The microstructure of the CNTs was characterized using SEM images recorded using a Carl Zeiss SUPRA 55VP FE-SEM at an acceleration voltage of 15 kV. The tortuosity of the CNTs was measured from an SEM image magnified by a factor of 500,000. The inner structure, inner diameter and wall number of the CNTs were statistically measured, and the pores of the open-ended membrane were observed from transmission electron microscopy (TEM) images recorded using a JEOL JEM-3000F high-resolution transmission electron microscope at an acceleration voltage of 300 kV. For the CNT purity measurements, Raman spectra were obtained using a confocal laser micro-Raman spectrometer equipped with a 532-nm laser source (LabRam 300, JY-Horiba) and a × 100 objective lens. Thermogravimetric analysis measurements (SETSYS 16/18) were performed over the temperature range from 20 to 800 °C at a heating rate of 5 °C min −1 . Functionalization at CNT tips was analysed by deconvolution of the C 1 s spectrum obtained by X-ray photoelectron spectroscopy (PHI 5000 VersaProbe II; Al-Kα source). Fabrication of the CNT wall membrane Vertically aligned CNTs were separated from the substrate. The CNTs were compressed by applying mechanical force in the direction perpendicular to the CNT axis ( Supplementary Figs 5 and 6 ). The mechanically densified CNTs were positioned on a commercial PTFE membrane (Millipore Fluoropore membrane filter, Model No. :FSLW04700, average pore size: 3 μm). The PTFE membrane filter is intrinsically hydrophobic. Therefore, the membrane was dipped in ethanol solution to make the membrane Hydrophilic and then dried in air. The PTFE membrane serves as a support layer for the CNTs. The CNT array on the PTFE membrane was surrounded by semicured highly viscous epoxy to clamp the CNT array under the high test pressure and to prevent test fluids from leaking through the side of the CNT array. The CNT array surrounded by the epoxy was then cured at room temperature for 24 h. The gel-like high-viscosity epoxy was obtained by curing the low-viscosity epoxy at room temperature for 24 h. Therefore, the epoxy did not permeate into the interstitial space between the CNTs (that is, the effective pore of the outer-wall CNT). Full curing of the epoxy required 48 h. The resulting membrane was the outer-wall CNT membrane used in the experiments. After the outer-wall membrane was fabricated, the outer-wall membrane was dipped into water and the outer-wall pores (interstitial space between the CNTs) were subsequently filled with water under vacuum. The permeability of the water-absorbed outer-wall membrane was measured using a dead-end filtration system ( Supplementary Fig. 7 ). The caps of the thermally purified outer-wall CNT membrane were opened using an RIE etcher (Oxford Instruments, RIE 80 plus) equipped with radio-frequency power. The radio-frequency power was set at 50 W, and the working pressure was ∼ 0.1 Torr in the chamber. During the RIE process, the flow rate of oxygen was set at 60 s.c.c.m. and the etching duration was 20 s. Antimicrobial tests of CNT membranes A carbenicillin-resistant derivative of P. aeruginosa PAO1 tagged with green fluorescent protein (Center for Biofilm Engineering, Montana State University) was used as a model bacterial strain. The feed solution was composed of 10 ml of 1/100 tryptic soy broth (Bacto, Franklin Lakes, NJ) and ∼ 1 × 10 7 CFU ml −1 of the initial bacterial concentration. Then, the outer-wall CNT membrane ( D f of 10), the CNT wall membrane and the commercial PSf UF membrane (UE4040, Woongjin Chemical Co., Korea) were immersed into the feed solution in six-well plates with stirring at 50 r.p.m. at 25 °C for 72 h. The feed solution was replaced with 10 ml of 1/300 tryptic soy broth solution every 24 h. Each sample was collected at 24, 48 and 72 h and then stained with a BacLight Live/Dead Bacterial viability kit (Molecular Probes, USA). After the samples were stained, bacterial adhesion and biofilm formation were observed using CLSM (Eclipse 90i, Nikon, Japan). More details are available elsewhere [33] . Pore size characterization of CNT membranes The pore size of the outer-wall VA CNT membrane was estimated by fitting to the hindered pore-flow solute transport model. This method is commonly used to determine the molecular weight cutoff of membranes for water treatment [37] , [38] , [39] . The Stokes radii for various dextran molecules were obtained from their molecular weights using the empirical equation [18] , [19] , [20] a =0.488 × M 0.437 , which was derived from the Stokes–Einstein relationship. From the rejection rate results ( Supplementary Table 1 ), the pore size was calculated using the Ferry–Renkin equation. Notably, >90% rejection was used for estimation of the pore size because the typical method for measuring the molecular weight cutoff is based on the 90% rejection of dextran solute [37] , [38] , [39] : where R is the rejection rate, a is the radius of the solute and r is the radius of the pore. How to cite this article: Lee, B. et al . A carbon nanotube wall membrane for water treatment. Nat. Commun. 6:7109 doi: 10.1038/ncomms8109 (2015).